Association ofCLEC16Awith human common variable immunodeficiency disorder and role in murine B cells Common variable immunodeficiency disorder (CVID) is the most common symptomatic primary immunodeficiency in adults, characterized by B-cell abnormalities and inadequate antibody response. CVID patients have considerable autoimmune comorbidity and we therefore hypothesized that genetic susceptibility to CVID may overlap with autoimmune disorders. Here, in the largest genetic study performed in CVID to date, we compare 778 CVID cases with 10,999 controls across 123,127 single-nucleotide polymorphisms (SNPs) on the Immunochip. We identify the first non-HLA genome-wide significant risk locus at CLEC16A (rs17806056, P =2.0 × 10 −9 ) and confirm the previously reported human leukocyte antigen (HLA) associations on chromosome 6p21 (rs1049225, P =4.8 × 10 −16 ). Clec16a knockdown (KD) mice showed reduced number of B cells and elevated IgM levels compared with controls, suggesting that CLEC16A may be involved in immune regulatory pathways of relevance to CVID. In conclusion, the CLEC16A associations in CVID represent the first robust evidence of non-HLA associations in this immunodeficiency condition. Common variable immunodeficiency (CVID) has a prevalence of ∼ 1 in 25,000 in European populations. Recurrent bacterial respiratory tract infections constitute the predominant clinical manifestation, but a subset of CVID patients also develops gastrointestinal manifestations and lymphoid hyperplasia. In addition, various forms of autoimmune disorders affect up to 25% of the patients, of which the most common is autoimmune thrombocytopenia [1] . The immunological hallmark of CVID is the B-cell defect with inability to produce adequate antibody responses, but patients also show other immunological abnormalities such as T-cell dysfunction, monocyte/macrophage hyperactivity and signs of low-grade systemic inflammation [2] . The focus of CVID genetics over the years has largely been to determine the presence of monogenic subtypes, leading to the identification of familial affection of a series of immunodeficiency genes, including CD19 (ref. 3 ), CD20 (ref. 4 ), CD81 (ref. 5 ), CR2 (ref. 6 ), ICOS [7] , LRBA [8] , PLCG2 (ref. 9 ), PRKCD [10] and TNFRSF13B [11] . However, most of the CVID cases are sporadic and although formal heritability estimates have not been made, a complex model of inheritance probably accounts for the majority of patients [12] . The human leukocyte antigen (HLA) haplotype association with CVID was found earlier by tissue typing [13] and a recent genome-wide association study in CVID further supports a complex genetic heritability in CVID, with common variants within the HLA complex associating with disease development [14] . To what extent common genetic variations outside this region contribute to CVID susceptibility is unknown. We hypothesize that the autoimmune comorbidity in CVID may occur on the basis of shared genetic susceptibility. We perform dense autoimmune risk loci genotyping on the Immunochip in 778 CVID cases and 10,999 controls, representing the largest CVID study panel investigated for genetic risk factors to date. We identify a novel non-HLA risk locus at CLEC16A and replicate the previously reported HLA associations at chromosome 6p21. In Clec16 knockdown (KD) mice, we found a reduced proportion of B cells and elevated IgM secretion, pointing to a role of CLEC16A in B-cell function of potential relevance to CVID and other CLEC16A associated conditions. 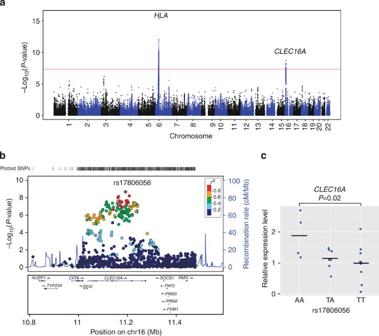Figure 1: The association statistics for CVID and the relative expression level of CLEC16A in different genotype groups. (a) A Manhattan plot of the Immunochip association statistics illustrating CVID susceptibility loci. SNP locations are plotted on thexaxis according to their chromosomal position. The negative log10ofP-values per SNP derived from the association analysis are plotted on theyaxis. The horizontal red line represents the genome-wide significance threshold ofP=5 × 10−8. (b) The regional association plot48for theCLEC16Alocus. The most associated SNP (rs17806056) is indicated by the purple dot, while the colours of the remaining SNPs indicate the LD with the index SNP, as shown in the colour legend. The light blue line shows the recombination rates (HapMap project49) and genomic positions are from genome build hg19. The plot was generated using software LocusZoom48. (c) The relative expression level of CLEC16A compared between CVID cases of different genotypes at rs17806056. The mRNA level of CLEC16A was assessed by quantitative reverse transcriptase–PCR and normalized to glyceraldehyde 3-phosphate dehydrogenase (GAPDH) control. The relative fold change (yaxis) was plotted against the genotype for SNP rs17806056 (xaxis). Each blue dot represents the average value of three measurements from each individual sample and the black line through the dots represents the mean level among each genotype group. The number of samples in each group isn=4 AA,n=7 TA andn=11 TT.P-value was determined by two-sidedT-test. A novel CVID susceptibility locus harbouring CLEC16A To systematically assess established autoimmune risk loci for associations in CVID, we genotyped 886 CVID cases and 11,552 controls of European ancestry from Sweden, Norway, Germany, United Kingdom and the United States ( Table 1 , Supplementary Table 1 and Supplementary Fig. 1 ), using the Immunochip, a targeted genotyping array with dense single-nucleotide polymorphism (SNP) coverage across 186 known disease loci from 12 immune-mediated diseases [15] . Following standard quality-control (QC) measures, a total of 123,127 SNPs with a minor allele frequency >1% from 778 cases and 10,999 controls remained available for analysis. Association testing was performed using logistic regressions with the first three principal components as covariates to adjust for population structure (residual genomic inflation factor λ =1.04) ( Supplementary Figs 2 and 3 ). Table 1 Overview of number of included patient and control panels before quality control, according to geography. Full size table On chromosome 16p13.13, we detected 22 genome-wide significant ( P <5 × 10 −8 ) SNPs spanning the CLEC16A locus in our logistic regression analysis. 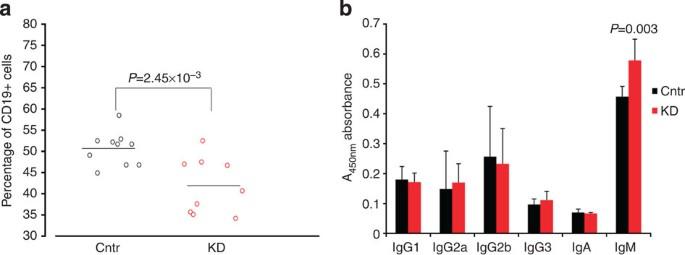Figure 2: The effect of inducible Clec16a KD in murine B cells. (a) Percentage of B cells (CD19+cells) from splenocytes of inducible Clec16a KD mice after tamoxifen treatment and the littermates treated with oil as a control in two independent experiments by fluorescence-activated cell sorting analysis. Data from the two experiments were combined. Black and red dots represent data from control (Cntr) andClec16aKD mice, respectively. The black lines through the dots represent the mean level among the ten control mice and nineClec16aKD mice, respectively. Two-sidedT-test was used to compare the percentage of CD19+cells betweenClec16AKD mice and control littermates. (b) Ig production from the supernatants of B cells, purified fromClec16AKD mice splenocytes, cultured with anti-mouse CD40 (100 ng ml−1) for 6 days. Data from two independent experiments were combined. Data are mean±s.d. of seven mice in each group. Two-sidedT-test was used to compare the level of each Ig subtype produced fromClec16AKD and control littermates. The most strongly associated SNP (rs17806056, P =2.0 × 10 −9 ) was located in intron 19 of CLEC16A ( Table 2 and Fig. 1a,b ). Fifteen additional imputed SNPs also showed genome-wide significance ( Supplementary Table 2 ). Conditioning on SNP rs17806056, significant associations of other CLEC16A SNPs were ablated, suggesting that the SNP is representative of a single association signal at CLEC16A . CLEC16A encodes a protein belonging to the C-type lectin-like domain family and is expressed in dendritic cells, natural killer cells and B cells [16] , [17] . Stratified analysis also suggested that CLEC16A variants may correlate with several clinical subtypes and immunological phenotypes in CVID (for example, lymphoid hyperplasia) and not just the autoimmune subtype ( Supplementary Table 3 ), although none of these associations were robust at the genome-wide significance level. Table 2 Genome-wide significant ( P <5 × 10 −8 ) associations detected by logistic regression analysis of 778 cases with CVID and 10,999 population controls. Full size table Figure 1: The association statistics for CVID and the relative expression level of CLEC16A in different genotype groups. ( a ) A Manhattan plot of the Immunochip association statistics illustrating CVID susceptibility loci. SNP locations are plotted on the x axis according to their chromosomal position. The negative log 10 of P -values per SNP derived from the association analysis are plotted on the y axis. The horizontal red line represents the genome-wide significance threshold of P =5 × 10 −8 . ( b ) The regional association plot [48] for the CLEC16A locus. The most associated SNP (rs17806056) is indicated by the purple dot, while the colours of the remaining SNPs indicate the LD with the index SNP, as shown in the colour legend. The light blue line shows the recombination rates (HapMap project [49] ) and genomic positions are from genome build hg19. The plot was generated using software LocusZoom [48] . ( c ) The relative expression level of CLEC16A compared between CVID cases of different genotypes at rs17806056. The mRNA level of CLEC16A was assessed by quantitative reverse transcriptase–PCR and normalized to glyceraldehyde 3-phosphate dehydrogenase (GAPDH) control. The relative fold change ( y axis) was plotted against the genotype for SNP rs17806056 ( x axis). Each blue dot represents the average value of three measurements from each individual sample and the black line through the dots represents the mean level among each genotype group. The number of samples in each group is n =4 AA, n =7 TA and n =11 TT. P -value was determined by two-sided T -test. Full size image We conducted quantitative real-time PCR on blood from CVID cases, to investigate whether there is any correlation between CLEC16A expression and the rs17806056 genotype. Statistically significant higher level of CLEC16A messenger RNA was detected in the AA group, which carries two copies of the minor allele, compared with the TT group ( Fig. 1c ). We did not find any significant difference in mRNA levels of the neighbouring SOCS1 or DEXI genes according to rs17806056 genotype status ( Supplementary Fig. 4 ). We further assessed annotations from the ENCODE [18] project for all CVID-associated SNPs within the 16p13.13 region ( Supplementary Table 4 ). Of note, several of the CVID-associated SNPs (rs36110069, rs35300161, rs2867880, rs7203459 and rs34972832) are predicted to affect binding sites for the GATA2 transcription factor where binding to SNP rs34972832 and neighbouring sequences is detected in the human K562 leukemia cell line [18] . GATA2 is also involved in different adult immunodeficiency state (monoMAC syndrome) [19] . Further studies are warranted to explore the relevance of these observations in vivo . Clec16 KD affects murine B cells Whereas CLEC16A is highly expressed in human B cells, a role of CLEC16A in these cells has not been established. Given the paramount importance of B-cell defects in CVID development, we explored the biological implications of Clec16a KD in murine B cells isolated from splenocytes. We detected a 54.4% (±8.4%) reduction of the total number of CD19 + B cells in the splenocyte population after induction of Clec16a KD using tamoxifen, when compared with non-tamoxifen-treated littermates (control group; P =6.25 × 10 −6 in two-sided T -test). In particular, the fraction of CD19 + B cells in splenocytes is reduced (17.4±5.0%, P =2.45 × 10 −3 in two-sided T -test) ( Fig. 2a and Supplementary Table 5 ). We did not detect significant differences in the fraction of CD27 + cells or for B-cell proliferation assaying (MTT (3-(4,5-dimethylthiazol-2-yl)-2,5-diphenyltetrazolium bromide)). However, B cells from Clec16a -deficient mice exhibited an altered immunoglobulin (Ig) profile as compared with control mice with increased levels of IgM ( P =0.003 in two-sided T -test), but no changes in serum levels of IgG and IgA ( Fig. 2b ). In sum, the supplementary murine Clec16a data suggest an impact of CLEC16A on B-cell function. Figure 2: The effect of inducible Clec16a KD in murine B cells. ( a ) Percentage of B cells (CD19 + cells) from splenocytes of inducible Clec16a KD mice after tamoxifen treatment and the littermates treated with oil as a control in two independent experiments by fluorescence-activated cell sorting analysis. Data from the two experiments were combined. Black and red dots represent data from control (Cntr) and Clec16a KD mice, respectively. The black lines through the dots represent the mean level among the ten control mice and nine Clec16a KD mice, respectively. Two-sided T -test was used to compare the percentage of CD19 + cells between Clec16A KD mice and control littermates. ( b ) Ig production from the supernatants of B cells, purified from Clec16A KD mice splenocytes, cultured with anti-mouse CD40 (100 ng ml −1 ) for 6 days. Data from two independent experiments were combined. Data are mean±s.d. of seven mice in each group. Two-sided T -test was used to compare the level of each Ig subtype produced from Clec16A KD and control littermates. Full size image Candidate gene association statistics In addition to the genome-wide significant CLEC16A locus, we also found six loci exhibiting suggestive evidence for association (5 × 10 −8 < P -value <5 × 10 −5 ; Supplementary Fig. 5 and Supplementary Table 6 ). Although replication in future study panels is required for formally establishing these loci ( FCRLA , EOMES , TNIP1 , TNFAIP3 , TNFSF11 and PTPN2 ) in CVID, prior probability for genuine association is enhanced by findings in other immune-mediated diseases ( Supplementary Table 6 ). Furthermore, SNPs at four genes previously suggested to be involved in familial CVID subtypes, CR2 , ICOS , MSH5 and TNFRSF13B , showed nominally significance association ( P <0.05) in the present analysis ( Supplementary Table 7 ). HLA-DQB1 associations In line with previous studies [14] we detected strong associations with SNPs within the HLA complex on chromosome 6p21, peaking at rs1049225 in the 3′ untranslated region of HLA-DQB1 ( P =4.8 × 10 −16 ; Table 2 , Fig. 1a and Supplementary Fig. 6 ). By stepwise conditional logistic regressions, we found that the association signal consists of multiple independent effects ( Supplementary Table 8 and Supplementary Fig. 7 ). We imputed classical HLA-A , HLA-C , HLA-B , HLA-DRB1 , HLA-DQB1 , HLA-DQA and HLA-DPB1 alleles ( Supplementary Table 9 ), revealing HLA-DQB1 associations with HLA-DQB1*02:01 and *05:03(risk alleles), as well as HLA-DQB1*06:02 and DQB1*06:03 (protective alleles). Further studies involving direct sequencing of all HLA class I and II loci and determination of their protein structure and peptide binding profiles are required to further explore the link between these HLA haplotypes and CVID development. It is noteworthy that for the present report, we found no statistical evidence for interaction between CLEC16A and the HLA-associated risk to CVID ( Supplementary Table 10 ). Autoimmune disease associations at the CLEC16A locus Genome-wide association studies have detected CLEC16A associations in multiple phenotypes ranging from prototypical autoimmune disorders (for example, type 1 diabetes [20] and primary biliary cirrhosis [21] ) via immune-mediated conditions driven by exogenous antigens (for example, celiac disease [22] and allergy [23] ) to suggestive associations ( P =1.8 × 10 −7 ) observed in selective IgA deficiency [24] . The majority of significant SNPs from these studies are trans -ethnic, localize to the same linkage disequilibrium (LD) block and are in high to moderate LD with the most strongly associated SNP within CLEC16A in the current study (rs17806056; Supplementary Table 11 ). The present study has demonstrated a potential role of CLEC16A in the pathogenesis of CVID by strong genetic associations and its involvement in murine B-cell function. Because of the prominent CLEC16A SNP associations in a variety of auto-immune diseases, several studies have been carried out to examine the biological function of CLEC16A. Its Drosophila homologue Ema has been found to localize to the endosomal and Golgi membranes [25] , [26] . Ema mutants show defects in lysosomal degradation and protein trafficking [25] . It is also essential for autophagosomal growth and autophagy processes [26] , which are of major importance for proper immune regulation, including regulation of inflammasome activation. CLEC16A is evolutionarily conserved and may rescue the Drosophila Ema mutant phenotypes [25] , [26] . Human CLEC16A has been reported to be abundantly expressed in dendritic cells, natural killer cells and B cells [16] , [17] . Zouk et al . [27] demonstrated, by using a human erythromyeloblastoid leukemia cell line, K562 cells, and human lymphoblastoid cell lines, that CLEC16A is localized with an endoplasmic reticulum marker, and that KD of CLEC16A did not affect T-cell co-stimulation. Recent murine data indicated that Clec16a is localized at endosomal membrane and forms a protein complex with Nrdp1, which is an E3 ubiquitin–protein ligase [28] . Clec16a may thus regulate mitophagy through the Nrdp1/Parkin pathway [28] . Adding to this existing knowledge, the present study has shown that CLEC16A may also be involved in B-cell function. Although we could not reproduce the complete CVID phenotype in Clec16a KD B cells, findings strongly suggest that CLEC16A, in combination with other dysregulated pathways, may contribute to the B-cell dysfunction observed in these patients. The relationship of CLEC16A expression and its genotype status has been investigated. We have previously shown that CLEC16A is differentially expressed based on the risk allele, reported with the protective minor allele showing a higher expression than the risk allele [20] , and a similar observation was made in the present study. The correlation is further complicated by the existence of three CLEC16A isoforms, which could lead to isoform-specific correlations. Examining the relative expression level of the long isoforms versus short isoform, a correlation with multiple sclerosis-associated SNP rs12708716 genotype status has been observed in human thymic tissues. However, no association was found when it was examined in whole blood [29] . Therefore, the effect of SNP genotype status on CLEC16A expression could be both isoform specific and cell-type/tissue-type dependent [30] . Furthermore, the sample size in each study is small and may be underpowered to detect a correlation. At this stage, although CLEC16A is a promising candidate gene to function in the pathogenesis of CVID as demonstrated in our study, we could not fully exclude the possibility that CVID-associated SNPs in CLEC16A introns are tagging other proximal genes, although we find this is unlikely. The identification of CLEC16A as a significant CVID risk locus reflects the notion that most genetic risk loci for immune-related diseases are pleiotropic. Significant overlap of risk loci between autoimmune disease and immune deficiency has also been found for those of rheumatoid arthritis [31] . The biological explanation of the overlap probably differs from locus to locus, but the overall interpretation is that of an imperfect relationship between clinical disease phenotyping and genetically determined pathophysiology. Importantly, the finding of CLEC16A associations in both autoimmunity, allergy and, as given by the present study, an immunodeficiency condition, characterized by impaired immune response to certain capsulated bacteria, is particularly interesting, as the mechanisms leading to persistent immune activation and autoimmunity in CVID is not clear. Our findings may suggest that altered function of CLEC16A could be ‘the missing link’ between immunodeficiency and immune action in CVID. The current identification of novel, highly robust CLEC16A associations in CVID raises conceptually novel opportunities for exploring mechanisms underlying the autoimmune co-morbidity and the chronic inflammation observed in CVID. Hypothetically, the CLEC16A -associated aspects of adult immunodeficiency states may reveal novel concepts for the basis of immune activation in autoimmunity. In conclusion, we have identified the first genome-wide significant non-HLA CVID risk locus at CLEC16A in the largest genetic study performed in this disease to date. CLEC16A has previously been linked to autoimmune disorders and the fact that Clec16a -deficient mice showed decreased number of B cells suggests that CLEC16A could represent a link between autoimmunity and immunodeficiency in CVID. Study subjects description Study subjects were recruited from five countries: Sweden, Norway, the United States, the United Kingdom and Germany ( Table 1 and Supplementary Table 1 ) The diagnosis of CVID was defined as decreased serum levels (>2 s.d.) of IgG, IgA and/or IgM, and exclusion of other forms of hypogammaglobulinemia according to the World Health Organization expert group on primary immunodeficiency and the International Union of Immunological Societies [32] , [33] . Controls were recruited from blood donors or population-based studies. The Swedish CVID cases ( n =93) were recruited at the Department of Laboratory Medicine, Division of Clinical Immunology and Transfusion Medicine, Karolinska University Hospital, Huddinge, Stockholm. The Swedish controls ( n =2,096) were part of a population based case–control study named Epidemiological Investigation of Rheumatoid Arthritis [34] . The CVID patients in the Norwegian panel ( n =112) were recruited from the Section of Clinical Immunology and Infectious Diseases at Oslo University Hospital Rikshospitalet, Oslo, Norway. DNA samples from healthy Norwegian controls ( n =1,405) were selected from the Norwegian Bone Marrow Donor Registry and the North-Trøndelag Health Study (HUNT). The CVID patients in the United States/United Kingdom panel ( n =330) were recruited from four locations: the Immunodeficiency Clinic at Mount Sinai Medical Center, New York, NY, the Division of Allergy, Immunology and Rheumatology, All Children’s Hospital, St Petersburg, FL, the Division of Allergy and Immunology at The Children’s Hospital of Philadelphia, PA, and the Department of Clinical Immunology in the Nuffield Department of Medicine, Oxford Radcliffe Hospital, UK. All the US/UK cases were genotyped at the Center for Applied Genomics, Children’s Hospital of Philadelphia, PA. The US controls ( n =1402) were recruited at the University of Michigan and genotyped at the Institute of Clinical Molecular Biology, Christian-Albrechts-University of Kiel (as part of the PAGE Immunochip data set [35] ). The German CVID cases ( n =351) were recruited at the Center for Chronic Immunodeficiency, University Hospital of Freiburg, and at the Clinic for Immunology and Rheumatology, Hannover Medical School, Hannover. DNA from 2,696 German healthy controls was obtained through the Northern German biobank PopGen [36] ( http://www.popgen.de ) and the University Hospital Schleswig-Holstein. Genotyping of these 2,696 controls was performed at the Institute of Clinical Molecular Biology, Christian-Albrechts-University of Kiel. One thousand nine hundred and twenty-four German controls were part of an independent population-based sample from the general population living in the region of Augsburg (Cooperative Health Research in the Region of Augsburg), southern Germany [37] , and were genotyped at the Helmholtz Center in Munich. One thousand and five hundred German controls were recruited from the population-based epidemiological Heinz-Nixdorf Recall study and genotyped at the Life and Brain Center at the University Clinic Bonn. Three hundred and fourteen individuals were of south German ancestry and were part of the control population Munich recruited from the Bavarian Red Cross and 215 individuals were recruited from the Charité-Univeristätsmedizin Berlin. These samples were genotyped at the University of Pittsburgh Genomics and Proteomics Core Laboratories. Respective regional ethics committees are listed for all sites that provided patients and/or controls to the study, all of which were approved: The regional ethical review board in Stockholm, The Regional Committees for Medical and Health Research Ethics South East (Norway) for Norwegian patients and The Regional Committee for Medical and Health Research Ethics Central (Norway) for the HUNT controls, Children's Hospital of Philadelphia Institutional Review Board, Mount Sinai School of Medicine Institutional Review Board, University of Oxford Institutional Review Board, University of South Florida Institutional Review Board, the University of Michigan Medical School Institutional Review Board, Ethikkommission der Universitätsklinik Freiburg, Ethik-Kommission der Medizinische Hochschule Hannover, Ethik-Kommission der Medizinischen Fakultät der Christian-Albrechts-Universität zu Kiel, Ethics committee of the University Hospital S.-H., Campus Kiel (Kiel University), Ethics committee of the Faculty of Medicine, Ludwig-Maximilians-University Munich, Germany, Ethikkommission der Bayerischen Landesärztekammer for the KORA controls, Ethikkommission der Universität Duisburg-Essen for HNR controls, Ethikkommission der Charité-Universitätsmedizin Berlin for Berlin Charite controls. Written informed consent for blood sample collection, processing and genotyping were obtained by all participants. Immunochip genotyping DNA samples were genotyped using the Immunochip, an Illumina iSelect HD custom genotyping array. This BeadChip was developed for highly multiplexed SNP genotyping and the SNP content of this array was mainly based on findings in ankylosing spondylitis, autoimmune thyroiditis, Crohn’s disease, celiac disease, IgA deficiency, multiple sclerosis, primary biliary cirrhosis, psoriasis, rheumatoid arthritis, systemic lupus erythematosus, type 1 diabetes and ulcerative colitis. Genotyping was performed according to Illumina protocols, with 4 μl of genomic DNA samples at 50 ng μl −1 , aliquoted to the corresponding wells of 96-well plates. The NCBI build 36 (hg19) map was used ( Illumina manifest file Immuno_BeadChip_11419691_B.bpm ) and normalized probe intensities were extracted for all samples passing standard laboratory QC thresholds. Genotype calling was performed with Illumina’s GenomeStudio data analysis software, the GenomeStudio GenTrain 2.0 algorithm and the cluster file generated by Trynka et al . [38] (based on the clustering of 2,000 UK samples and subsequent manual re-adjustment of cluster positions). All CVID cases from Norway, Sweden and Germany were genotyped at the Institute of Clinical Molecular Biology in Kiel, Germany. The US/UK cases were genotyped at the Center for Applied Genomics, the Children’s Hospital of Philadelphia, USA. Quality control Sample QC measures included sample call rate, overall heterozygosity, relatedness testing and other metrics: samples with a SNP call rate<98% ( n =309) as well as heterozygosity outliers ( n =15), defined as beyond 5 s.d. of the mean, were excluded from analysis. Duplicate samples ( n =37) and cryptically related samples (PI_HAT ⩾ 0.1875; n =199) were identified through identity-by-state calculations with PLINK [39] . For each pair of duplicate or related samples, the sample with the highest SNP call rate was kept in the data set. Finally, removal of population outliers (non-Caucasians; n =101) was performed based on principal component analysis of population heterogeneity, which is described below in detail as ‘Principal component analysis’. In the SNP-based QC SNPs with a call rate <98%, with a minor allele frequency <1% and markers that deviated from Hardy–Weinberg equilibrium test ( P -value<10 −5 ) in the controls or SNPs with significant different genotyping rate between cases and controls ( P <1 × 10 −5 in Fisher’s exact test) were removed. Applying the QC procedures described above resulted in 778 CVID cases and 10,999 controls available for association analysis. Principal component analysis Principal component analysis was conducted once to identify ethnic outliers and once again to generate covariates to control for population stratification. For the first analysis, we used HapMap samples as a reference set and 13,001 uncorrelated SNPs that passed the above QC criteria and are present in both our Immunochip data set and HapMap data set, which were LD pruned such that no pair of SNPs had r 2 >0.2 and excluding problematic GC/AT SNPs and X- and Y-chromosomes. PLINK was used for LD pruning and exclusion of SNPs. All samples that did not cluster with the European samples were excluded. After removal of ethnicity outliers, second principal component analysis was performed within the remaining Immunochip samples to resolve within-Europe relationships. No population stratification in the remaining samples was observed. Principal component analyses were performed using EIGENSTRAT [40] version 4.0. Association analysis For case–control association testing, logistic regression with PLINK was performed using the first three principal components from the EIGENSTRAT analysis as covariates, which are sufficient to control for potential population stratification as determined by the genomic inflation factor. Subphenotype analysis was similarly conducted via logistic regression. Step-wise conditional association analysis was performed by including the most strongly associated SNP in the previous step as a covariate. Post-hoc power assessment showed over 99% power to detect genome-wide significant association at the HLA SNP rs1049225 (odds ratio (OR)≈1.75) with 778 cases and 14-fold number of controls, and ∼ 83% power for the CLEC16A SNP, rs17806056 (OR≈1.5; Supplementary Fig. 8 ). SNP imputation and association testing For the CLEC16A locus on chromosome 16, haplotype pre-phasing was performed using SHAPEIT [41] , [42] version 2. Genotype imputation was conducted using the IMPUTE2 (refs 43 , 44 ) package. The 1000 Genomes Phase I integrated variant set was used as reference panel and data were downloaded from the IMPUTE2 website ( http://mathgen.stats.ox.ac.uk/impute/data_download_1000G_phase1_integrated.html ). After imputation, the SNPTEST v2 package was used to perform association analysis on the imputed genotypes. Missing data likelihood score test, implemented in SNPTEST [43] v2, was employed to take imputation uncertainty into account. The first three principal components were included in the model as covariates. SNPs with low quality, with info score<0.8 or with Hardy–Weinberg equilibrium test P -value<10 −6 were excluded. Power analysis Power analysis was conducted using software Power for Genetic Association [45] , with the following settings: Genetic Model=Co-dominant (1 df) SNP analysis; R 2 =1; Disease prevalence=0.00004; Marker allele frequency=Disease allele frequency=0.75; Effective degree of freedom=123,127; α =0.05 and control to case ratio=14. Relative risk was set at 1.5, 1.75 and 2, to generate three power curves. Animals All animal studies were approved by the Institutional Animal Care and Use Committee of the Children’s Hospital of Philadelphia. To generate Clec16a loxP mice, a 15.3-kb DNA fragment containing Clec16a exons 2–4 and flanking intronic sequence was retrieved from C57BL/6 mouse genomic DNA and subcloned into plasmid FLSniper (Ozgene) that contains an FRT-flanked PGK-driven Neomycin cassette for negative selection. One loxP site was inserted upstream of exon 3, while a second loxP site was placed downstream of exon 3. The linearized targeting vector was electroporated into B6 ES cells and clones that survived selection were screened for homologous recombination by Southern blot analysis. Targeted clones were injected into C57BL/6-derived blastocysts that were then transferred to pseudopregnant females. Male offspring were mated to C57BL/6 females and ES cell-derived offspring were identified by PCR-based genotyping. Mice harbouring the targeted insertion of the two loxP sites in the Clec16a gene locus were then crossed to the Flpo Deleter line (mouse Strain: 129S4/SvJae-Gt(ROSA)26Sortm2(FLP*)Sor/J; The Jackson Laboratory) to achieve deletion of the FRT-flanked Neomycin cassette. Clec16a loxP mice were mated to UBC-Cre-ER-LBD-tg mice (inducible cre recombinase driven by the human ubiquitin C promoter), to generate UBC-Cre-Clec16a loxP mice. To generate experimental groups, UBC-Cre-Clec16a loxP male mice were treated with tamoxifen (for Clec16a KD) or oil (control group). Tamoxifen (MP Biomedical) was prepared at a concentration of 20 mg ml −1 in 10% ethanol and 90% corn oil (Sigma). Four-week-old male mice received 1 mg of tamoxifen at 24-h intervals for 5 consecutive days by gavage. Control group of mice were receiving an equal volume of corn oil alone. After tamoxifen treatment was finished, mice were aged an additional 2 weeks before evaluation. Quantitative real-time PCR The total RNA was extracted from human blood using Trizol (Ambion, Life Technologies) and converted to complementary DNA with High Capacity RNA-to-cDNA Kit, following the manufacturer’s protocols (Applied Biosystems). Briefly, 1 ml of Trizol was mixed to 50 μl of whole blood, followed by 200 μl of chloroform. The mixture was centrifuged at 12,000 g for 15 min at 4 °C. The upper aqueous phase (containing RNA) was purified with RNAeasy kit (Qiagen). Quality of RNA was assessed by Agilent Bioanalyzer. Fluorescence-based real-time PCR was performed in 10 μl of reaction mixture, using cDNA, TaqMan Universal Master Mix and 20 × FAM-MGB TaqMan assays (Applied Biosystems): Hs00322376_m1 (CLEC16A), Hs00360234_m1 (DEXI), Hs00705164_s1 (SOCS1) and Hs02758991_g1 (glyceraldehyde 3-phosphate dehydrogenase). Relative gene expression was normalized to glyceraldehyde 3-phosphate dehydrogenase. All PCR runs were performed on ViiA 7 Real Time PCR System using ViiA7 RUO software v1.2.2 (Life Technologies). Flow cytometry Single-cell suspensions from murine spleens (10 6 cell per test) were stained with fluorochrome-conjugated monoclonal antibodies in a single tube containing anti-mouse CD19-Alexa Fluor 647 (BioLegend 115522), IgD-Alexa Fluor 488 (BioLegend, 405718), IgM-Brilliant Violet 421 (BioLegend 406517) and CD27-PE (BioLegend 124209) antibodies (1:20 dilution) for 30 min at 4 °C. Cell-associated fluorescence was assessed with an LSR-II flow cytometer and analysed using FACSDiva software (both BD). Two independent experiments were conducted, comparing the percentage of CD19 + cells (B cells) from splenocytes between inducible Clec16a KD mice after tamoxifen treatment and the littermates treated with oil as a control. Data were combined together and B-cell percentage was compared via two-sided T -test. Naïve B-cell proliferation and Ig synthesis Naive B cells from splenic cell suspensions were negatively selected using EasySep Mouse B-cell Enrichment Kit, following the manufacturer’s instructions (StemCell). Purified B cells were suspended in RPMI containing 10% fetal bovine serum, L -glutamine and 50 μM β-mercaptoethanol (complete medium). For Ig synthesis, naive B cells (10 6 cell per ml) were cultured in complete medium alone, with lipopolysaccharide (20 μg ml −1 ; Sigma-Aldrich) or with anti-mouse CD40 (100 ng ml −1 ; Pharmingen). Supernatants were collected after 6 days and analysed for various Ig production by Pierce ELISA Mouse mAb Isotyping Kit, following the manufacturer’s instructions (Thermo Scientific). Proliferation was measured using Cell Proliferation Kit I (MTT), following the manufacturer’s instructions (Roche). For proliferation, aliquots of 10 5 B cell in 100 μl of complete medium alone, or in the presence of lipopolysaccharide (20 μg ml −1 ) or anti-mouse CD40 (100 ng ml −1 ), were cultured in a 96-well flat-bottom plate for 48 h, then the MTT labelling reagent was added to a final concentration 0.5 mg ml −1 followed by overnight incubation with the solubilization solution. Proliferation was assessed by measuring the absorbance using a microplate (ELISA) reader. HLA analyses Conditional analysis did not demonstrate evidence for independent association signals at the HLA-DQBI locus. Imputation of classical alleles at HLA class I and II loci was performed using SNP2HLA with a reference panel consisting of 5,225 unrelated individuals collected by the Type 1 Diabetes Genetics Consortium [46] . To further explore the HLA class I and HLA class II associations with CVID, HLA allele frequencies between cases and controls at a two-digit level were analysed. The effect size of the association was measured with OR and the confidence interval for the OR was calculated directly from the 2 × 2 table using the Woolf’s formula [47] . Western blot analysis For western blot analysis, lysis of splenocytes was performed with NP40 lysis buffer (Invitrogen). Proteins were separated on 4–12% NuPAGE Bis-Tris gels in MOPS SDS running buffer and transferred overnight onto nitrocellulose membranes (Invitrogen). The membranes were blocked in 3% BSA and cut in half. The upper half of the membranes was incubated with rabbit anti-CLEC16A polyclonal antibody (Abgent, AP6983c) at 1:1,000 dilution and the lower half of the membranes was probed with mouse anti-β-Actin monoclonal antibody (Abcam, ab6276) at 1:1,000 dilution. The membranes were washed, incubated with corresponding secondary antibody for 1 h and washed again; bound antibody was detected with WesternBright ECL chemiluminescence detection system (Advansta). Band intensities were measured using Image J software (NIH Shareware). Representative western blot for Clec16a in splenocytes of Clec16a KD and control mice is shown in Supplementary Fig. 9 . How to cite this article: Li, J. et al . Association of CLEC16A with human common variable immunodeficiency disorder and role in murine B cells. Nat. Commun. 6:6804 doi: 10.1038/ncomms7804 (2015).